Anomalous magnetoresistance in the spinel superconductor LiTi2O4 LiTi 2 O 4 is a unique compound in that it is the only known spinel oxide superconductor. The lack of high quality single crystals has thus far prevented systematic investigations of its transport properties. Here we report a careful study of transport and tunnelling spectroscopy in epitaxial LiTi 2 O 4 thin films. An unusual magnetoresistance is observed which changes from nearly isotropic negative to prominently anisotropic positive as the temperature is decreased. We present evidence that shows that the negative magnetoresistance likely stems from the suppression of local spin fluctuations or spin-orbit scattering centres. The positive magnetoresistance suggests the presence of an orbital-related state, also supported by the fact that the superconducting energy gap decreases as a quadratic function of magnetic field. These observations indicate that the spin-orbital fluctuations play an important role in LiTi 2 O 4 in a manner similar to high-temperature superconductors. LiTi 2 O 4 (LTO) is an oxide superconductor with a spinel crystal structure [1] . It was discovered in early 1970’s by Johnston et al . [2] , and it has the superconducting transition temperature T c of 11 K (ref. 1 [1] ). Although its T c can be described by band-structure calculations using the McMillan formula with a weak electron-phonon coupling constant ( λ el-ph ∼ 0.6; refs 3 , 4 ), an enhanced density of states or an equivalently larger coupling constant has been unveiled from specific-heat [5] , [6] and magnetic susceptibility measurements [7] . Other measurements like nuclear magnetic resonance [8] , point contact Andreev reflection spectroscopy [9] , and resonant inelastic soft-x-ray scattering [10] have revealed the significance of d – d electron correlations. It is naturally expected that the correlations play a role in the microscopic mechanism for its superconductivity. Moreover, in contrast to perovskite oxides, LTO has a cubic symmetry with the space group of Fd3m , where the lithium and titanium cations are located at the tetrahedral 8 a and octahedral 16 d sites [7] , respectively. On one hand, the t 2g sub-band of Ti is in high degree of degeneracy, remaining in a narrow d -band metal with significant electron–electron interaction [8] , [11] . On the other hand, the Ti sublattice, in mixed valences of Ti 3+ and Ti 4+ , is frustrated and favours short-range spin ordering [12] . Therefore, it is interesting to see whether spin-orbital fluctuations also play a role in superconductivity in LTO, akin to the perovskite-type high T c superconductors [13] , [14] . However, the development of an understanding of this system has been hampered by the lack of sample reproducibility and the availability of single crystals or high quality thin films [1] , [7] , [15] . Recently, high quality epitaxial LTO thin films were successfully grown by pulsed laser deposition [16] , [17] , thus opening the door for systematic experiments on LTO. In this paper, we present results of transport and tunnelling studies on single crystalline-like epitaxial LTO thin films. The suppression of the superconducting energy gap as a quadratic function of magnetic field, and an anomalous crossover of magnetoresistance from prominently anisotropic positive to nearly isotropic negative with increasing temperature have been observed for the first time. In addition to the extracted key parameters from the combined tunnelling and transport measurements, a full picture of LTO has emerged: the data suggest the presence of spin-orbit scattering/spin fluctuations below ∼ 100±10 K and an orbital-related state below T ch ∼ 50±10 K. We propose a theoretical model to account for the relation between the superconducting energy gap and the magnetic field. Charge transport data and tunnelling spectra The (00 l )-Oriented LTO thin films were epitaxially grown on (00 l )-oriented MgAl 2 O 4 substrates by pulsed laser deposition. Our LTO films consistently display T c of 11±0.25 K with narrow transition widths of <0.5 K. We have found that different films have different residual resistivity ratios (RRR). The films were patterned into Hall bars to carry out Hall and normal resistivity measurements. Tunnelling spectroscopy was performed where Pt–Ir tips were used to make point contacts in the out-of-plane axis direction ( c -axis, perpendicular to the film plane) of LTO [18] . 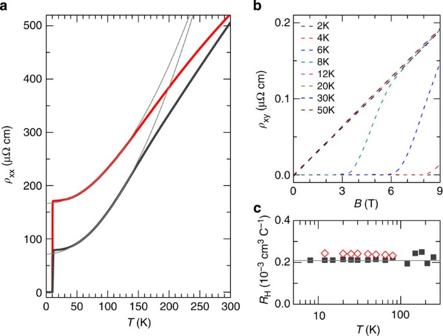Figure 1: Resistivity and Hall behavior of LiTi2O4thin films. (a)ρxx(T) of two samples. They have similar resistivity (∼500 μΩ cm) at room temperature, and the sameTcof 11 K, but different residual resistivity ratios (RRR): RRR∼6.25 for Sample L1 (black curve) and∼3 for the Sample L2 (red curve). The resistivity curve from 40 to 120 K can be fit byρ=ρ0+AT2(grey lines). (b) The Hall resistivity is proportional to the magnetic field at different temperatures, and all theρxy(B) curves overlap in the normal state (only data on Sample L1 are shown here), suggesting a simple one band-structure and a temperature-independent Hall coefficient. Note that at very low temperatures, the magnetic field is not sufficient to suppress the superconductivity (B⊥abplane). (c) Hall coefficient versus temperature for both samples (L1: solid symbols. L2: open symbols). Though the two samples show different RRR, their Hall coefficient values are very close to each other. AssumingRH=1/(ne), we find a hole concentration of∼3 × 1022cm−3, which is almost constant over the entire measured temperature range. Figure 1a shows the resistivity versus temperature curves for samples with two different RRR ratios: 6.25 and 3 for samples L1 and L2, respectively. L1 and L2 have similar resistivity values at room temperature and the same T c . The normal state resistivity of both samples can be fitted to a curve consistent with the Fermi liquid behaviour, ρ = ρ 0 + AT 2 (grey lines) from 40 to 120 K with residual resistivity ( ρ 0 ) of ≈71 μΩ cm for L1 and ≈166 μΩ cm for L2. The deviation from the Fermi liquid behaviour at low temperatures is caused by an enhanced electron–electron interaction as discussed below. By sweeping the magnetic field perpendicular to the film surface ( B ⊥ in-plane ( ab plane)) at fixed temperatures, the Hall resistivity, that is, , has been extracted. ρ xy data for different temperatures are plotted in Fig. 1b , where V y is the Hall voltage obtained by subtracting the transverse voltage in negative field from that in positive field, and t is the thickness of the film. In the normal state, the Hall resistivity is always proportional to the magnetic field, positive and temperature independent, strongly suggesting the presence of one type of charge carriers (holes) and a simple electronic band structure. The charge carrier concentration is calculated assuming a parabolic band structure, that is, the Hall coefficient . L1 and L2 have almost the same hole concentration of ∼ 3 × 10 22 cm −3 ( Fig. 1c ), indicating that the different RRRs are likely caused by the difference in mobility values. Figure 1: Resistivity and Hall behavior of LiTi 2 O 4 thin films. ( a ) ρ xx ( T ) of two samples. They have similar resistivity ( ∼ 500 μΩ cm) at room temperature, and the same T c of 11 K, but different residual resistivity ratios (RRR): RRR ∼ 6.25 for Sample L1 (black curve) and ∼ 3 for the Sample L2 (red curve). The resistivity curve from 40 to 120 K can be fit by ρ = ρ 0 + AT 2 (grey lines). ( b ) The Hall resistivity is proportional to the magnetic field at different temperatures, and all the ρ xy ( B ) curves overlap in the normal state (only data on Sample L1 are shown here), suggesting a simple one band-structure and a temperature-independent Hall coefficient. Note that at very low temperatures, the magnetic field is not sufficient to suppress the superconductivity ( B ⊥ ab plane). ( c ) Hall coefficient versus temperature for both samples (L1: solid symbols. L2: open symbols). Though the two samples show different RRR, their Hall coefficient values are very close to each other. Assuming R H =1/( ne ), we find a hole concentration of ∼ 3 × 10 22 cm −3 , which is almost constant over the entire measured temperature range. Full size image The point contact measurements were carried out on L1 before it was patterned into a Hall bar for transport measurements. As described by the Blonder, Tinkham and Klapwijk (BTK) model [19] , the tunnelling regime is achieved for Z >1, where Z represents the tunnelling barrier height and the Fermi velocity mismatch [20] . The differential conductance spectrum shows a clear temperature and field-dependent coherence peak. The normalized differential conductance spectra with and without applied magnetic field are shown in Fig. 2a–c as a function of bias voltage (see Supplementary Note 1 for normalization procedure). The normalized experimental curves were fitted using a modified BTK model with a complex energy E ′= E+i Γ (ref. 21 ). The broadening Γ term, which takes into account sample inhomogeneity and a finite quasi-particle lifetime by scattering, is temperature independent in zero field, but application of magnetic field has been found to lead to an additional pair-breaking factor [22] , which in effect is akin to an enhanced Γ (ref. 23 ). 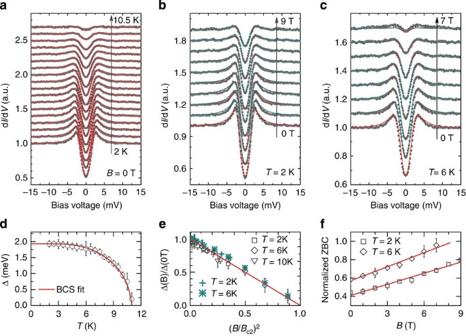Figure 2: Temperature- and field-dependent tunnelling spectroscopy curves and the superconducting energy gap of LTO films. (a) Normalized differential conductance versus bias voltage from 2 to 10.5 K (ΔT=0.5 K) in zero field. Experimental data are fitted with a modified BTK model with a constant broadening Γ term (red lines), and are vertically shifted above the 2 K curve for clarity. (b,c) Normalized differential conductance versus field from 0 to 9 T at 2 K, and from 0 to 7 T at 6 K (ΔB=1 T,B⊥abplane). Experimental data (grey circles) are fitted with a modified BTK model with an increasing Γ asBis increased (red lines), and also with the two-channel model (cyan lines). Data in fields are vertically shifted. (d) Temperature-dependent energy gap values, Δ(T), are obtained from the BTK fits: 2Δ/kBTc=4 is obtained, indicating a medium-coupling BCS-like superconductor. (e) Normalized energy gap (Δ(B)/Δ(0T)) decreases as (B/Bc2)2in the superconducting state, and can be scaled for different temperatures. In-field measurements were carried out atT=2, 6 and 10 K (open symbols extracted from modified BTK fittings with an increasing Γ and cross symbols from the two-channel model). (f) The normalized zero bias conductance (symbols) at 2 and 6 K shows a linear dependence on the magnetic field (red straight fitting line). The error bars ind–frepresent the s.e. in the fit to the data. Figure 2: Temperature- and field-dependent tunnelling spectroscopy curves and the superconducting energy gap of LTO films. ( a ) Normalized differential conductance versus bias voltage from 2 to 10.5 K (Δ T =0.5 K) in zero field. Experimental data are fitted with a modified BTK model with a constant broadening Γ term (red lines), and are vertically shifted above the 2 K curve for clarity. ( b , c ) Normalized differential conductance versus field from 0 to 9 T at 2 K, and from 0 to 7 T at 6 K (Δ B =1 T, B ⊥ ab plane). Experimental data (grey circles) are fitted with a modified BTK model with an increasing Γ as B is increased (red lines), and also with the two-channel model (cyan lines). Data in fields are vertically shifted. ( d ) Temperature-dependent energy gap values, Δ( T ), are obtained from the BTK fits: 2Δ /k B T c =4 is obtained, indicating a medium-coupling BCS-like superconductor. ( e ) Normalized energy gap (Δ( B )/Δ(0T)) decreases as ( B / B c2 ) [2] in the superconducting state, and can be scaled for different temperatures. In-field measurements were carried out at T =2, 6 and 10 K (open symbols extracted from modified BTK fittings with an increasing Γ and cross symbols from the two-channel model). ( f ) The normalized zero bias conductance (symbols) at 2 and 6 K shows a linear dependence on the magnetic field (red straight fitting line). The error bars in d – f represent the s.e. in the fit to the data. Full size image Fitting parameters and superconducting energy gap Several key points can be made from the fitting of our tunnelling spectra. First, the Z value of our Pt–Ir/LTO junction is ∼ 2.4, which is independent of temperature and field. Second, zero-field spectra give a constant Γ of ∼ 0.94 meV ( Supplementary Fig. 2 ), but data in field have to be fitted with an increasing Γ as the field is increased ( Supplementary Fig. 3 ). Third, the temperature dependence of the superconducting energy gap can be fitted well with the BCS theory ( Fig. 2d ), and the observed 2Δ 0 / k B T c =4 (Δ 0 =1.93 meV) is consistent with previous reports [6] , [9] , indicating that LTO is a medium-coupling BCS superconductor. Moreover, a simple relation of Δ( B , T )/Δ(0T, T ) ∼ −[ B / B c2 ( T )] [2] , can be used to scale the field-dependent energy gap at different temperatures, for example, T =2, 6, 10 K ( Fig. 2e ). Accordingly, B c2 can be extracted from the point contact spectra with B c2 (2K) ∼ 16 T. We also employed a two-channel method derived from the BTK model to fit our experimental data [24] . In this method, the pair-breaking effect by field is considered as a normal channel (N) superposed onto the superconducting channel (S). Assuming the differential conductance to take the form G( h )= h r G N +(1− h r )G S with h = B / B c2 , the normalized differential conductance in field should obey the polynomial form , where is obtained from the BTK model with a constant Γ. The best fitting requires r =2. We note that this value is consistent with those used to fit data for point contacts with other superconductors such as Nb, Mo 3 Sb 7 and Dy 0.8 Y 0.2 Rh 4 B 4 (ref. 24 ). In this case, the relation, Δ( B ) ∼ − B 2 emerges again, and the Δ values extracted from the two fitting methods are similar ( Fig. 2e ). To the best of our knowledge, none of the existing theoretical models can account for the quadratic relation. When B is close to B c2 , the Maki formula [25] can be analytically expressed as , where represents the averaged energy gap taking into account the effect of vortices, and Ψ 2 is the first derivative of the digamma function with A the pair-breaking parameter proportional to B when B ⊥ ab plane [26] , but this does not lead to a quadratic field dependence of the superconducting energy gap. Theoretical model We note, however, that if there exists an additional anisotropy axis, which breaks the intrinsic symmetry of the system, for example, orbital ordering or a background nematicity, Δ( B ) ∼ − B 2 can arise. To simplify the discussion without loss of generality, we assume that the superconducting order parameter is a three-component vector, Δ=(Δ x , Δ y , Δ z ). The isotropic gap is then equal to the modulus of this vector: Δ 0 = (ΔΔ) 1/2 =(Δ x 2 +Δ y 2 +Δ z 2 ) 1/2 . In zero field, the orientation of the local spin of the Cooper pair changes in real space, while the value of the gap does not change. Therefore, the average magnetic moment of Cooper pairs vanishes, that is, < Δ(r)> = 0 . However, in magnetic field B , the magnetic moments of Cooper pairs can be partially polarized, and therefore the susceptibility χ can develop a paramagnetic component. Thus, we have χ super = χ para + χ dia , where the last term is the conventional diamagnetic susceptibility of a superconductor. The first term χ para should be a function of the magnetic moments of the Cooper pairs, which contributes to the symmetry invariants. There are in general three symmetry invariants here. The first one is just ΔΔ, the second one is ΔB . The additional anisotropy axis, for example, orbital ordering or background nematicity associated with some vector b results in another invariant as Δb . In the vicinity of the phase transition, we can use the Taylor expansion to obtain: In using this expression, the total free energy of the superconductor in the lowest order with superconducting order parameter can be written in the form: Minimization of the free energy with respect to Δ will give the expression Δ( B )= (ΔΔ) 1/2 = (− α /2 β ) 1/2 − δbB 2 /2| α | where α , β and δ are the parameters of the Ginzburg–Landau expansion, and b is the modulus of the vector b (See Supplementary Note 4 for details). This represents the first plausible explanation giving rise to the relation, Δ( B ) ∼ − B 2 . As for the origin of the symmetry breaking, which gives rise to the vector b in LTO, we propose that there is an onset of orbital ordering, which takes place in LTO below a transition temperature T ch , arising from orbital degeneracy of t 2g sub-band [27] , [28] . We would like to point out that although this relation has not been carefully examined previously, we also observe it in some cuprates, namely, electron-doped (Nd,Ce) 2 CuO 4 and (Pr,La,Ce) 2 CuO 4 ( Supplementary Fig. 4 ), indicating the presence of a similar symmetry breaking ordering in these compounds. We believe other ordering mechanisms such as spin stripes or charge density wave may also lead to a symmetry breaking resulting in the vector b . The electronic nematicity has been widely discussed in hole-doped cuprates [29] , [30] and Fe-based superconductors [31] , [32] as a competing order to the superconductivity. The exact nature of the ordering in electron-doped cuprates is beyond the scope of the present work [33] , but the discovered quadratic relation is perhaps not uncommon across different types of superconductors. On the other hand, we note that the relation from the Maki formula is observed in superconductors without symmetry breaking, for example, Δ 2 ( B ) ∼ − B or − B 2 for Zn (ref. 34 ) and Δ 2 ( B ) ∼ − B (Ba,K)BiO 3 (ref. 35 ). It would therefore be of broad interest to investigate the possible occurrence of the quadratic relation in other superconductors also: it can possibly serve as a signature underpinning different mechanisms leading to intrinsic symmetry breaking, which results in the presence of an additional anisotropy axis. Zero bias conductance The normalized zero bias conductance (ZBC) at 2 and 6 K shows a linear dependence on the magnetic field (see Supplementary Note 3 for calculation details), indicating a linear increase of the vortex density with uncorrelated vortices ( Fig. 2f ). Such a relation has been reported in systems such as Bi 2 Sr 2 CaCu 2 O 8+ δ overdoped with intercalating HgBr 2 molecules [36] and in nanosized Pb islands on a silicon wafer [37] . The departure from linearity in-field-dependent ZBC has previously been observed in MgB 2 (ref. 38 ) and YNi 2 B 2 C (ref. 39 ), associated with the fact that they are multiband superconductors. In the Ca 2- x Na x CuO 2 Cl 2 ( x =0.14), the field dependence scales as B log B , suggested to be an indication of a dirty d -wave superconductor [40] . Previous specific heat experiments have suggested that LTO is an s -wave superconductor [6] . Thus, based on the lack of departure from the linearly dependent ZBC, we conclude that LTO is not likely to be a multiband superconductor. Calculated key physical quantities Combining the transport and tunnelling data, we were able to extract key parameters for LTO. The Ginzburg–Landau coherence length, the size of the vortex core in type II superconductor is estimated to be . The mean free path of l =1.8 nm is deduced from the Drude model , where the Fermi wave vector k F =(3 π 2 n ) 1/3 =0.96 Å −1 . Since l<ξ GL , the BCS coherence length of ξ BCS =14.9 nm is calculated from the dirty limit relation, . We then calculate the Fermi velocity from the formula, ξ BCS =ħ v F / π Δ, and arrive at an effective mass of m */ m 0 =8.11 (with m 0 being the free electron mass), and the density of states at the Fermi level is found to be N( E F )=0.96 states per eV atom. We compared these parameters to those obtained from previous reports on LTO. Only T c and ξ GL values have been previously reported on thin films [16] , and the other quantities were from the magnetic susceptibility [7] , Andreev reflection [9] and specific heat [6] measurements on polycrystalline samples. As seen in Table 1 , the values obtained in the present work are consistent with those from previous reports. We note that in polycrystalline samples, the grain boundaries prevent accurate calculations from the transport measurements due to boundary scattering, but the parameters could be extracted from heat capacity and susceptibility data. These values indicate that the nearly free electron model can capture the main physics of the LTO system. Table 1 Comparison of physical parameters of LiTi 2 O 4 to values from previous work. Full size table Field direction dependence of magnetoresistivity In the normal state, we observe an anomalous MR behaviour. 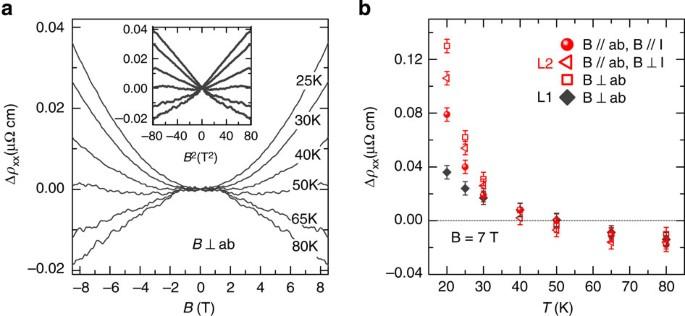Figure 3: Temperature dependence of magnetoresistivity. (a) The transverse magnetoresistivity withB⊥abplane, Δρxx=ρxx(B)−ρxx(0T), changes from negative to positive as temperature is decreased. The crossover temperature is∼50±10 K. The positive magnetoresistivity is proportional toB2as seen in the inset, whereas the negative MR is not. (b) Magnetoresistivity at 7 T plotted against the temperature. The dark and red symbols are for samples L1 and L2, respectively. The magnetic field was applied along three different directions, that is,B//abplane (B//I,B⊥I) andB⊥abplane. The error bars are maximum data noise in determining the magnetoresistivity. The negative magnetoresistivity is nearly isotropic, whereas the positive magnetoresistivity shows unambiguous anisotropy. Figure 3a illustrates the field-dependent MR in sample L1 when B ⊥ ab plane. The MR gradually decreases from positive to negative with increasing temperature, and a crossover is observed at 50±10 K. In the inset of Fig. 3a , the MR is plotted as B 2 . The positive MR is proportional to B 2 , whereas the negative MR is not. In the case of B ⊥ ab plane, both orbital and spin effects can contribute to MR, and in order to discern the different contributions additional measurements were carried out where the field was also applied in the film plane with B // I (parallel to current) and B ⊥ I (normal to current). In Fig. 3b , the temperature dependence of MR is plotted for both L1 (grey symbols) and L2 (red symbols). The negative MR is nearly independent of the field directions, but the positive MR displays unambiguous anisotropy, that is, MR ( B ⊥ ab plane) >MR ( B // ab plane, B ⊥ I ) >MR ( B // ab plane// I ). Moreover, the MR changes its sign when B // I , as seen in Fig. 4a . The first derivative of ρ xx ( T ) in zero field (symbols) starts to deviate from the Fermi liquid behaviour (d ρ xx /d T ∼ T ) at roughly the same range of temperature as seen in Fig. 4b , indicating the presence of an enhanced electron–electron interaction. Figure 3: Temperature dependence of magnetoresistivity. ( a ) The transverse magnetoresistivity with B ⊥ ab plane, Δ ρ xx = ρ xx ( B )− ρ xx (0T), changes from negative to positive as temperature is decreased. The crossover temperature is ∼ 50±10 K. The positive magnetoresistivity is proportional to B 2 as seen in the inset, whereas the negative MR is not. ( b ) Magnetoresistivity at 7 T plotted against the temperature. The dark and red symbols are for samples L1 and L2, respectively. The magnetic field was applied along three different directions, that is, B // ab plane ( B //I, B ⊥ I) and B ⊥ ab plane. The error bars are maximum data noise in determining the magnetoresistivity. The negative magnetoresistivity is nearly isotropic, whereas the positive magnetoresistivity shows unambiguous anisotropy. 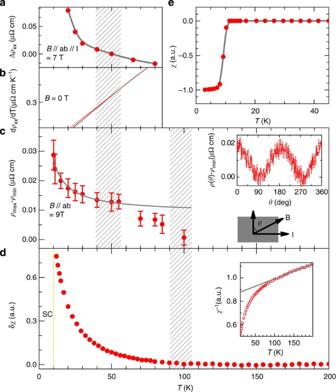Figure 4: Magnetoresistivity and susceptibility features of LiTi2O4thin films. (a) Temperature-dependent longitudinal magnetoresistivity (B//abplane//I), Δρxx=ρxx(B)−ρxx(0T), is replotted to demonstrate the crossover temperature (also seeFig. 3b). (b) dρxx/dTin zero field. It deviates from the Fermi liquid behaviour, dρxx/dT∼T(grey line), at lower temperatures. (c) Twofold symmetry of in-plane (abplane) resistivity, whereρmax(θ=90°) andρmin(θ=0°) are found from plots such as indicated in the inset. The inset shows a typical twofold symmetry at 30 K and 9 T againstθ, which is the angle between the normal direction to current and the field. The error bars are maximum data noise as seen in the inset. (d) The susceptibility with field cooling (1,000 Oe,B//abplane) shows a Curie–Weiss behaviour at high temperature (see insetχ−1(T)). We plot the residual susceptibilityδχas a function of temperature after subtracting the paramagnetic contribution. Theδχstarts to increase below 100±10 K, coincident with the starting temperature of the twofold symmetry of in-plane resistivity. (e) The susceptibility with zero-field cooling shows a good superconducting screening signal, suggesting our LTO films are of high quality. The shading areas around 100 K and 50 K represent the uncertainties in defining the starting point of the anisotropic AMR and the abrupt increase, respectively. Full size image Figure 4: Magnetoresistivity and susceptibility features of LiTi 2 O 4 thin films. ( a ) Temperature-dependent longitudinal magnetoresistivity ( B // ab plane//I), Δ ρ xx = ρ xx ( B )− ρ xx (0T), is replotted to demonstrate the crossover temperature (also see Fig. 3b ). ( b ) d ρ xx /d T in zero field. It deviates from the Fermi liquid behaviour, d ρ xx /d T ∼ T (grey line), at lower temperatures. ( c ) Twofold symmetry of in-plane ( ab plane) resistivity, where ρ max ( θ =90°) and ρ min ( θ =0°) are found from plots such as indicated in the inset. The inset shows a typical twofold symmetry at 30 K and 9 T against θ , which is the angle between the normal direction to current and the field. The error bars are maximum data noise as seen in the inset. ( d ) The susceptibility with field cooling (1,000 Oe, B // ab plane) shows a Curie–Weiss behaviour at high temperature (see inset χ −1 ( T )). We plot the residual susceptibility δχ as a function of temperature after subtracting the paramagnetic contribution. The δχ starts to increase below 100±10 K, coincident with the starting temperature of the twofold symmetry of in-plane resistivity. ( e ) The susceptibility with zero-field cooling shows a good superconducting screening signal, suggesting our LTO films are of high quality. The shading areas around 100 K and 50 K represent the uncertainties in defining the starting point of the anisotropic AMR and the abrupt increase, respectively. Full size image Such transport data collectively point to the presence of a phase transition or crossover with a characteristic temperature T ch of ∼ 50±10 K. As discussed above, we believe orbital ordering results in the relation, Δ( B ) ∼ − B 2 . Thus, we associate T ch with the onset of an orbital-related state such as orbital ordering or nematicity (see Supplementary Note 4 ). If the LTO system indeed has such a symmetry breaking feature, it should also manifest itself in the anisotropy of the in-plane angular-dependent magnetoresistivity (AMR) measurements, and a twofold symmetry would be expected, similar to the case of iron arsenide superconductors [41] . We indeed observe a twofold AMR in LTO ( Fig. 4c ). Note that a strong enhancement in amplitude of the twofold symmetry takes place below T ch : we associate this with the orbital-related ordering. On the other hand, we find that the starting temperature of the twofold AMR is ∼ 100±10 K, far above the T ch . Temperature dependence of magnetic susceptibility To understand this unusual behaviour, we also measured the temperature-dependent susceptibility in zero field and field cooling. The χ ( T ) in zero-field cooling data shows a clear screening effect due to superconductivity <11 K ( Fig. 4e ). In-field cooling, we find that the residual susceptibility, δχ ( T ), found by subtracting a paramagnetic component from the χ ( T ), starts to increase below 100±10 K ( Fig. 4d ), corresponding to the same temperature where the twofold symmetry emerges. The amplitude of the twofold symmetry exhibits an abrupt increase at T ch =50±10 K. We, thus, attribute the twofold AMR to two sources: one related to a spin interaction starting at a higher temperature (100±10 K), and the other associated with an orbital effect (discussed below) becoming pronounced below T ch =50±10 K. Our findings, thus far, can be summarized in the following three points: (1) With decreasing temperature, the magnetic susceptibility increases and deviates from the Curie–Weiss behaviour <100±10 K, while the in-plane AMR starts to show a twofold symmetry and the magnetoresistivity is negative in field; (2) At T ch ∼ 50±10 K, the sign of magnetoresistivity changes to positive and the twofold symmetry becomes more prominent, where we also observe deviation from the Fermi liquid behaviour; (3) Below 11 K, LTO enters the superconducting state, where the superconducting energy gap decreases as a function of B 2 . Generally, MR can result from charge, orbital or spin interactions, as well as interactions among them [42] . The observed constant Hall coefficient and smooth temperature evolution of the c -axis lattice parameter ( Supplementary Fig. 8 ) preclude the presence of charge density waves, which normally influences the Hall coefficient [43] . The mean free path of the ‘clean’ sample (L1) is 1.84 nm in the zero-temperature limit, which is only about two unit cells of the LTO lattice. Therefore, a grain boundary effect is unlikely to have a dominant role in the MR behaviour. The combination of points (2) and (3) above supports an orbital effect as the origin of the positive anisotropic MR below 50±10 K, which introduces the additional anisotropic axis in the system used in the theoretical model. The temperature at which the twofold AMR at 100±10 K emerges corresponds to the temperature where the increase in antiferromagnetic-like spin correlation takes place (and where the Curie–Weiss fitting intercepts the temperature axis at negative value), indicating that the negative MR is associated with a spin interaction. We note that in La 2- x Ce x CuO 4 thin films, antiferromagnetism (AFM) has been identified as the main cause of a twofold symmetry of AMR and a negative MR [44] , while in Fe-based superconductors the anisotropy of in-plane charge transport was found to be associated with a nematic order [41] . Though the spinel structure is different from the perovskite one, we believe it is not unreasonable to link the appearance of a twofold symmetry of AMR at 100±10 K to local AFM spin correlations, and the sudden enhancement at 50±10 K to an orbital related state. In antiferromagnetic metals, a sign change in MR is expected theoretically at the Neel temperature due to the s–d electron interaction [45] . However, this idea is based on long range AFM, and the change in sign from negative to positive is to be accompanied by a discontinuous jump in MR. This is in contrast to the observation in LTO, where there is no discontinuous jump. Moreover, the LTO system has a frustrated Ti sublattice containing equal numbers of Ti 3+ and Ti 4+ , and thus a long range AFM ordering is unfavourable [12] . The emergence of short-range AFM ordering has been reported in V-doped LTO by nuclear magnetic resonance [11] and in LiV 2 O 4 by inelastic neutron scattering [46] . Note that the AMR measurements cannot be used to tell whether the AFM is static or dynamic. It is possible that local spin fluctuations are responsible for the negative MR. We consider an alternative explanation due to the effect of spin-orbit coupling. When the orbital ordered (nematic) state is destroyed at T > T ch , some ‘fluctuating’ islands may have a finite lifetime and serve as additional (magnetic) scattering centres for the electron transport. When the magnetic field is applied, some of these islands disappear and the resistivity decreases. This is exemplified in thin metallic Mg films covered with small controlled quantities of a magnetic ion such as Fe or a heavy ion with large spin-orbit coupling such as Au: the magnetoresistance changes its sign from negative to positive on experiencing an increase in the number of spin-orbit scattering centres [47] . Perhaps a similar mechanism is at work in LTO. In conclusion, detailed properties of superconducting LTO were investigated for the first time in high quality thin films. Many properties are consistent with previous work on polycrystalline samples: we observe one type of charge carrier and a value consistent with a medium-coupling BCS superconductor. The main physics can be captured by the nearly free electron model. However, we find two new and distinct features in this system. In the superconducting state, a scaling law, Δ ( B ) ∼ − B 2 at T < T c , is extracted from our point contact spectra. This behaviour had not been predicted by any previous theory. In the normal state, an anomalous MR, which crosses over from nearly isotropic negative MR to an anisotropic positive MR with decreasing temperature, is observed. The anisotropic positive MR likely originates from the enhanced electron–electron interaction due to the orbital related ordering below T ch ∼ 50±10 K. The negative MR occurring at 100±10 K possibly stems from the suppression of spin-orbit scattering or local spin fluctuations. We present a new theoretical model based on the proposal that there is orbital ordering in the superconducting state to account for the relation Δ( B ) ∼ − B 2 . The fact that this relation is also observed in other materials ((Nd,Ce) 2 CuO 4 and (Pr,La,Ce) 2 CuO 4 ) points to the broader applicability of the model developed here in understanding underlying interactions in different types of superconductors. How to cite this article : Jin, K. et al . Anomalous magnetoresistance in the spinel superconductor LiTi 2 O 4 . Nat. Commun. 6:7183 doi: 10.1038/ncomms8183 (2015).